Flooding disturbances increase resource availability and productivity but reduce stability in diverse plant communities The natural world is increasingly defined by change. Within the next 100 years, rising atmospheric CO 2 concentrations will continue to increase the frequency and magnitude of extreme weather events. Simultaneously, human activities are reducing global biodiversity, with current extinction rates at ~1,000 × what they were before human domination of Earth’s ecosystems. The co–occurrence of these trends may be of particular concern, as greater biological diversity could help ecosystems resist change during large perturbations. We use data from a 200–year flood event to show that when a disturbance is associated with an increase in resource availability, the opposite may occur. Flooding was associated with increases in productivity and decreases in stability, particularly in the highest diversity communities. Our results undermine the utility of the biodiversity–stability hypothesis during a large number of disturbances where resource availability increases. We propose a conceptual framework that can be widely applied during natural disturbances. Biodiversity is thought to ensure ecosystem functioning and stability in a changing world [1] , [2] , [3] . The positive relationship between biodiversity and stability is often attributed to the insurance hypothesis: higher diversity communities contain more species with unique strategies for withstanding environmental perturbation [4] , [5] , [6] , [7] , [8] , [9] , [10] , [11] . However, there is currently little consensus about the consistency of this trend across ecosystems and types of disturbances [4] , [6] , [8] , [9] , [10] , [11] . Understanding these relationships on a mechanistic level is becoming increasingly important, as climate change is increasing the occurrence and severity of these extreme perturbations globally [12] . Importantly, the biodiversity–stability hypothesis is predicated on the assumption that environmental perturbation will have a predominantly negative effect on productivity [4] , [6] , [8] , [13] ( Fig. 1c,d ). The majority of terrestrial biodiversity–stability studies have assessed disturbances, such as drought and warming, which result in both physiological stress and a reduction in resources. These types of disturbances consistently result in net productivity declines [4] , [8] , [13] . Furthermore, only when productivity is reduced, do our predictions about biodiversity—stability relationships make sense. Stability indicates smaller negative deviations from the baseline and a positive biodiversity–productivity slope reflects increased biodiversity, increased productivity, and increased stability ( Fig. 1g ) [4] , [6] . 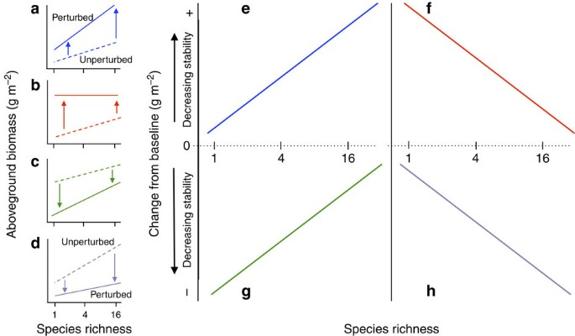Figure 1: Theoretical biodiversity–stability relationships. Potential changes in productivity before and after a disturbance are displayed in smaller panels (a–d). Initial conditions in this conceptual framework all reflect positive biodiversity–productivity relationships (see ref.9for alternatives). The consequent changes in biomass (often referred to as resistance or recovery) are displayed in the larger panel on the right. Biodiversity–stability predictions are based on disturbances that constitute stress and loss of productivity (c,d,g,h). However, if a disturbance constitutes a resource enrichment (a,b), we may expect increased productivity, but decreased stability in the highest diversity plots (e). Depending on the presence of negative selection effects, we may also expect smaller productivity increases in the highest diversity plots and therefore greater stability (f) or greater productivity losses in the highest diversity plots and therefore reduced stability (h). Figure 1: Theoretical biodiversity–stability relationships. Potential changes in productivity before and after a disturbance are displayed in smaller panels ( a – d ). Initial conditions in this conceptual framework all reflect positive biodiversity–productivity relationships (see ref. 9 for alternatives). The consequent changes in biomass (often referred to as resistance or recovery) are displayed in the larger panel on the right. Biodiversity–stability predictions are based on disturbances that constitute stress and loss of productivity ( c , d , g , h ). However, if a disturbance constitutes a resource enrichment ( a , b ), we may expect increased productivity, but decreased stability in the highest diversity plots ( e ). Depending on the presence of negative selection effects, we may also expect smaller productivity increases in the highest diversity plots and therefore greater stability ( f ) or greater productivity losses in the highest diversity plots and therefore reduced stability ( h ). Full size image In a system increasingly defined by change [14] , it is unrealistic to expect disturbance to have exclusively negative effects on productivity [15] . To date, no experimental or observational study has explicitly explored how biodiversity–stability predictions should change for the large number of disturbances (either pulse or press [8] ) that involve a resource enrichment (N deposition, CO 2 enrichment, fire, and flooding). In these instances, we would predict net increases in productivity following a disturbance due to increased resource availability [16] , [17] and comparatively more growth in higher diversity communities where resources are more limiting ( Fig. 1a ). For example, there may be instances (such as nitrogen deposition) where a resource enrichment causes physiological stress for some plants [18] , but drives a community–wide increase in productivity, particularly in higher diversity communities [17] . Mechanistically, this is because higher diversity communities include more species with unique resource needs and unique resource acquisition strategies: resource consumption is therefore more comprehensive, resource availability is generally lower [17] , [19] , and resource influxes can be used more readily [17] . These scenarios demonstrate the counterintuitive case where increased biodiversity leads to increased productivity ( Fig. 1a ), but decreased stability ( Fig. 1e ). In fact, diversity can lead to decreased stability when productivity either increases ( Fig. 1e ) or declines ( Fig. 1h ): this pattern simply reflects stronger effects on productivity at higher relative to lower diversity communities. However, the distinction between the two is important, as one reflects a greater capacity of the community to take advantage of resource influxes ( Fig. 1e ), and one reflects a greater mathematical probability for loss when productivity is higher to begin with ( Fig. 1h ). This difference highlights an inherent and important tension between productivity and stability. For the instances where disturbance increases productivity over the previous baseline, is stability a useful indicator of overall ecosystem health? Here we report on a natural 200–year flood event [20] that occurred in June 2013 in a well–established grassland biodiversity experiment in Jena, Germany. We show that flooding increased the availability of resources (namely water and nitrate), and this led to increased productivity. Higher diversity communities were most capable of taking advantage of such resource influxes and thus were more productive than before. However, increased productivity constituted a large deviation from baseline productivity, and thus higher diversity communities were also less stable. We emphasize the importance of understanding changes in productivity, when it may be at odds with stability. Response to mild flooding We found that when flooding severity was low, biomass production immediately following the flood (July 2013) in the highest diversity plots was higher than it had been since 2010 (compared with May and August 2010–2012, Fig. 2 , Supplementary Fig. 2 , Table 1 , Supplementary Table 1 ). This large increase in plant growth was likely due to increased water availability ( Fig. 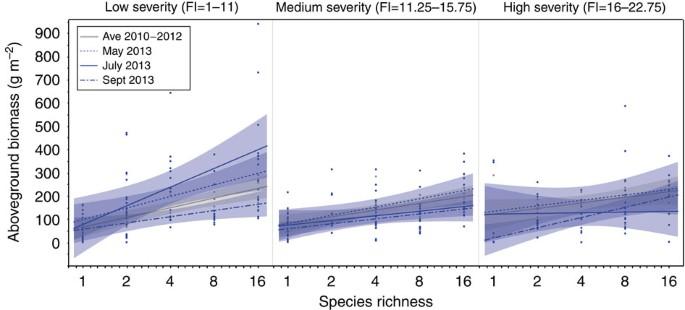Figure 2: Aboveground biomass over time. Living aboveground biomass (AGB) was measured in May 2013, early July 2013 (immediately following the flood), and September 2013 (2 months after the flood) and compared with AGB measurements from May and August of previous years (2010–2012) using a mixed effects statistical model. Values from previous years are averaged for comparison here, though explicit values were used in analyses. Flood intensity (FI) levels were determined for display by dividing plots into three equally sized groups (Nlow=25,Nmedium=25,Nhigh=26). AGB was highest in higher diversity/low flood severity plots in July 2013. Shaded areas represent 95% confidence intervals. 3a , Table 2 ), which led to increased growth in higher diversity plots after the flood waters receded ( Supplementary Fig. 3 , Supplementary Table 2 ). By September 2013, in the least flooded plots these patterns continued, due likely to a continuation or ‘legacy’ effect of the positive July 2013 growth patterns through to September 2013 ( Supplementary Fig. 4 ). Figure 2: Aboveground biomass over time. Living aboveground biomass (AGB) was measured in May 2013, early July 2013 (immediately following the flood), and September 2013 (2 months after the flood) and compared with AGB measurements from May and August of previous years (2010–2012) using a mixed effects statistical model. Values from previous years are averaged for comparison here, though explicit values were used in analyses. Flood intensity (FI) levels were determined for display by dividing plots into three equally sized groups ( N low =25, N medium =25, N high =26). AGB was highest in higher diversity/low flood severity plots in July 2013. Shaded areas represent 95% confidence intervals. Full size image Table 1 Plant community responses to flooding. 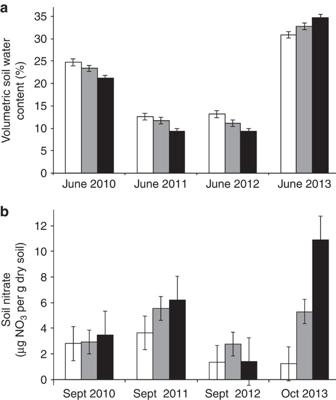Figure 3: Volumetric soil water content and soil nitrate over time. Volumetric soil water content (%) at 20 cm depth was measured during the final 2 weeks of June 2010, 2011, 2012, and 2013. Low flooding severity plots are indicated with white bars (n=25), grey bars represent medium severity plots (n=25), and the highest flooding severity plots are indicated with black bars (n=26). Comparisons were made in June to assess the direct role of the flood, which happened in June. Soil moisture was highest in June 2013 and increased with increasing flooding severity (a). Soil nitrate increased with increasing flooding severity in 2013 (b). For all comparisons, values were binned into three flooding severity classes (equal sample sizes in each) for display purposes only. Error bars represent s.e. of binned groups. Full size table Figure 3: Volumetric soil water content and soil nitrate over time. Volumetric soil water content (%) at 20 cm depth was measured during the final 2 weeks of June 2010, 2011, 2012, and 2013. Low flooding severity plots are indicated with white bars ( n =25), grey bars represent medium severity plots ( n =25), and the highest flooding severity plots are indicated with black bars ( n =26). Comparisons were made in June to assess the direct role of the flood, which happened in June. Soil moisture was highest in June 2013 and increased with increasing flooding severity ( a ). Soil nitrate increased with increasing flooding severity in 2013 ( b ). For all comparisons, values were binned into three flooding severity classes (equal sample sizes in each) for display purposes only. Error bars represent s.e. of binned groups. Full size image Table 2 Resource and microbial responses to flooding. Full size table Response to severe flooding In contrast, at higher levels of flooding severity (more than 11 days of whole plot submergence), the increase in soil water availability during the flood acted as a stress axis, likely related to reduced oxygen availability (see Supplementary Methods ) [21] , and did not further increase plant growth ( Supplementary Fig. 3 ). In fact, when flooding intensity was highest (>16 fully submerged days), biomass production immediately following the flood (July 2013) was slightly lower (though not significantly different) than in previous years, and positive biodiversity–productivity relationships disappeared ( Fig. 2 ). The loss of the positive biodiversity–productivity relationship (present in all previous years of the experiment) when flooding was severe indicates higher levels of stress, resulting in complete cessation of growth and loss of biomass for the entire community ( Supplementary Fig. 5 ) [22] , and thus no potential for insurance effects reflected in community biomass. This may be due to the degree of physiological strain experienced (compared with drought events) or to the strategy of flood tolerance that was employed (some species may survive, but stop growing, via a ‘sit and wait’ strategy [21] ). Surprisingly, though this was one of the strongest natural flooding events in 200 years [20] , biodiversity–productivity relationships in the most severely flooded plots returned to levels seen in previous years by September 2013. This pattern was particularly true in the highest diversity communities ( Supplementary Fig. 8 ). This unexpected rapid rebound was likely related to increased nutrient availability associated with the flood. Specifically, microbial biomass at the site was ~1.5 × higher after the rains began in May 2013 than in previous years, and continued at this higher level on average through September 2013 ( Table 2 ). This paired with greater inputs of dead organic material ( Supplementary Fig. 5 ) led to increased soil nitrate after the flood in the plots that experienced the most severe flooding ( Fig. 3b , Table 2 ). Consequently, in September 2013, growth in the highest diversity plots that experienced the most severe flooding, likely rebounded due to increased nitrate availability and an increased ability to take advantage of resource inputs in higher diversity communities ( Supplementary Fig. 6 , Supplementary Table 3 ) [17] . Most plants may have lost biomass during the flood, but survived the event [22] , and thus been able to regrow using the nutrients recycled following the recession of the flood waters. Species diversity losses Finally, we found that species were not lost from most of the plots and species evenness was not strongly affected by the flood, except when flooding severity was very high (almost 17 days with complete plot submergence, Supplementary Fig. 7 , Table 1 ). In these cases, Shannon diversity index was reduced most in the highest diversity plots in July 2013, and the loss of species and/or evenness remained through September 2013 ( Supplementary Fig. 7 ). This pattern was reflected in an average of 3–4 species lost from each of the highest diversity plots, where most of these species were small herbs (70% of cases) or legumes (30% of cases). This type of biodiversity loss may prime the system for further loss of ecosystem functions in the future [23] . Implications for stability Our results demonstrate the previously unreported case where increased productivity is at odds with increased stability ( Fig. 1c ). Specifically, we found that decreased stability ( Fig. 4g,i ) of higher diversity communities was sometimes due to increased biomass production ( Fig. 4a,f ). Flooding increased the availability of resources and higher diversity communities could more readily take advantage of such a resource enrichment. These patterns differ strikingly from past work on disturbances such as drought, where resources are depleted (not enriched) and productivity consistently declines [4] , [6] , [13] , [24] . When the resource enrichment that we report here was outweighed by the severity of flooding stress [15] , higher diversity communities were also less stable ( Fig. 4i ), but due to decreases in biomass production ( Fig. 4c ). Longer term resilience of communities experiencing severe flooding reflected the third case ( Fig. 1g ) where productivity declined overall, and higher diversity communities were more stable ( Supplementary Fig. 8 ). These results demonstrate the lack of a mechanistic link between diversity, productivity, and stability in general: stability reflects both productivity maintenance and a lack of ability to capitalize on resource gains. Furthermore, past work that has focused primarily on stability [11] , [24] or exclusively on the slope of the resistance relationship [4] , [6] , [10] , [13] may not have captured the far–reaching implications of reductions in resistance or stability that resulted from increases in productivity. 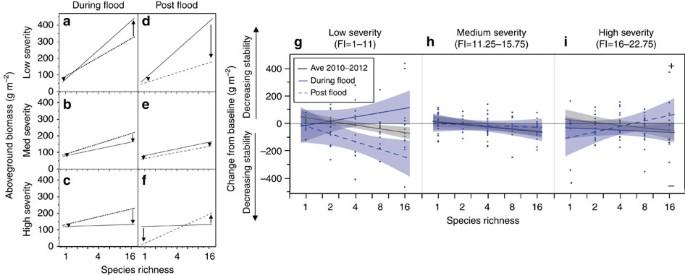Figure 4: Temporal stability over time. Temporal stability was measured as absolute change in biomass over time. We averaged seasonal stability measures for 2010–2012 (within year stability averaged over the 3 years prior to the flood) and compared with the temporal stability during the flood (May 2013–July 2013) and the temporal stability following the flood (July 2013–September 2013) using a mixed effects statistical model (n=76 per time interval). Biomass in higher diversity plots that experienced a small amount of flooding increased during the flood (a), and this resulted in decreased stability (g). As flooding severity increased, this turned into a net loss of biomass, particularly at higher levels of diversity (c). This was reflected in decreased productivity and decreased stability of the highest diversity plots (i). This same negative biodiversity–productivity–stability relationship held true for community recovery post flood in the lowest severity plots (d). However, recovery in the highest severity plots was positive for more diverse communities and slightly negative for less diverse communities (f), resulting in a positive relationship between biodiversity and productivity, but decreased stability at both low and high diversity (i). Intermediate levels of flooding for both resistance (b) and recovery (e) resulted in little relationship between diversity and stability (h). Figure 4: Temporal stability over time. Temporal stability was measured as absolute change in biomass over time. We averaged seasonal stability measures for 2010–2012 (within year stability averaged over the 3 years prior to the flood) and compared with the temporal stability during the flood (May 2013–July 2013) and the temporal stability following the flood (July 2013–September 2013) using a mixed effects statistical model ( n =76 per time interval). Biomass in higher diversity plots that experienced a small amount of flooding increased during the flood ( a ), and this resulted in decreased stability ( g ). As flooding severity increased, this turned into a net loss of biomass, particularly at higher levels of diversity ( c ). This was reflected in decreased productivity and decreased stability of the highest diversity plots ( i ). This same negative biodiversity–productivity–stability relationship held true for community recovery post flood in the lowest severity plots ( d ). However, recovery in the highest severity plots was positive for more diverse communities and slightly negative for less diverse communities ( f ), resulting in a positive relationship between biodiversity and productivity, but decreased stability at both low and high diversity ( i ). Intermediate levels of flooding for both resistance ( b ) and recovery ( e ) resulted in little relationship between diversity and stability ( h ). Full size image Climate change is expected to increase the occurrence and magnitude of extreme weather events in the future [12] , with large–scale implications for humans [25] . Our findings demonstrate the hitherto unavailable example of how plant diversity may buffer against such changes during a real–world flood. For the first time, we can address the simultaneous importance of both disturbance–related stress and disturbance–related resource availability. For the large number of disturbances that increase the availability of resources (fire, flood, CO 2 enrichment, and N deposition), future work should explore how productivity in higher diversity communities changes following the disturbance. We emphasize that diversity must be maintained at high levels, not for the sake of stability per se , but for the combined ability to take advantage of resource influxes when they do occur, and buffer against loss of species and ecosystem functions when environmental stress is severe [23] . Summary of the approach The Jena Biodiversity Experiment is located on a Central European mesophilic floodplain on the banks of the Saale River and described in detail in previous papers [26] , [27] . In summary, the current experiment consists of 78 experimental plots of 30 m 2 with plant species richness levels ranging from plant monocultures to 16–species mixtures. While there is much variation among past studies in the calculation of stability [4] , [6] , [11] , [24] , we assessed stability responses using absolute change in aboveground live biomass over time. We calculated this stability metric for the period during the flood (often referred to as resistance, but see Supplementary Fig. 1 ), for the two–month period following the flood (often referred to as initial recovery) and for the entire season before and after the flood (often referred to as resilience) and compared these values to average seasonal changes for the standard growing season in previous years (May–August 2010–2012). We also measured flooding duration and severity in each plot and subdivided flooding severity levels into three equally sized groups (for display only, low=1–11 days, medium=11.25–15.75 days and high=16–22.75 days). Flood conditions Rainfall in May 2013 in Jena was ~150 mm, constituting >25% of annual precipitation at the site that year. Overall the flood affected the entire Elbe River Basin and much of Europe [25] and was one of the largest natural flooding events in the past two centuries [20] . Temperatures at the site were cooler than average (2002–2012) leading up to and during the flood (12.3 °C in May 2013 compared with a 10–year average of 13.5 °C±1.1 °C and 16.4 °C in June 2013 compared with an average of 17.2 °C±1.1 °C) and slightly warmer than average immediately after the flood (19.7 °C in July 2013 compared with an average of 18.9 °C±1.1 °C). The flood lasted for a total of 24 days at the site (30 May–24 June) and led to anaerobic soil conditions (redox potentials ranging from −121 to 193 mV, Supplementary Methods ). Due to small topographical differences among the plots in the experiment (<1 m), there was variation in the duration of flooding and the proportion of each plot that was flooded. This variation was well–distributed across the diversity gradient. To assess the importance of flood severity, we quantified the proportion of each plot that was flooded for each of the 24 days of the flood and calculated a flooding index . For the purposes of display only, we split these flooding severity levels into three categories (minimum number necessary to display and examine linear trends) that represent three equally sized groups ( N low =25, N medium =25, N high =26). This allowed for visual display and examination of three–way interactions. Site description The Jena Experiment was established in 2002 using 60 grassland species from four functional groups (grasses, legumes, tall herbs and small herbs) that are commonly occurring in ecologically similar areas near the field site [26] . Species were randomly assigned to each of the five levels of biodiversity: 1, 2, 4, 8, and 16 species (60 species mixtures were established as well, but replicated four times, which means they were not replicated across the range of flooding severity levels, and thus were not used in these analyses). All plant diversity levels were replicated 14–16 times ( N =78). All plots were weeded regularly since the establishment of the experiment and are mown twice per year to mimic typical management of Central European grasslands [26] . Beginning in 2010, the plot size was reduced from 100 to 30 m 2 , and we utilized the biomass data from after the plot–reduction for the purposes of a consistent comparison. Aboveground biomass was measured in spring (late May) and summer (late August) of each year using two randomly placed 20 × 50 cm clip strips (2010–2012) at the same time as mowing. Clip strips were harvested, sorted to species, dried, and weighed. In 2013, aboveground biomass was sampled using clip strips on 29 May (immediately prior to the flood), sampled and mowed on 7 July (5 weeks after normal mowing and immediately following the flood), and sampled and mowed again on 7 September (4 weeks after normal mowing). Biomass harvests (mowing) in 2013 were delayed by ~4 weeks (compared with previous years) due to the flooded conditions in June. For all clip strips for all sampling dates, dead plant matter in the 20 × 50 cm areas was also collected and weighed separately. Realized species richness of each plot on each sampling date was determined by counting the species that were found in each clip strip in each plot. Shannon diversity index was calculated using the biomass proportions in each clip strip. We also measured soil moisture (at 20 cm depth), soil microbial biomass (pooled sample of three soil cores per plot; 0–5 cm soil depth), and soil nitrate in all plots (0–15 cm soil depth) in parallel to the repeated samplings of the plant community. Soil water Volumetric soil water content was measured at 10–20 cm in the centre of every plot once per week for the duration of the field season (April–September 2010–2013) pending appropriate weather (the measurement cannot be taken while it is raining). Measurements were taken using a frequency domain reflectometry probe inserted into a PVC access tube (PR2, Delta T Devices Ltd, Cambridge, UK). During the June 2013 flood, weather conditions and standing water made it impossible to measure soil moisture in all plots on all days. To compare soil moisture at the height of the flood with soil moisture in previous years, soil moisture was measured on 20 June (on 84% of the plots; the plots not measured were also those that were most flooded) and 24 June (100% of the plots) and averaged to calculate a June 2013 average. Due to the flooding of soils and ongoing rain, this value is still likely an underestimation of actual soil moisture over the course of the flood. This June 2013 average was compared with the average of the final 2 weeks of June in previous years (2010–2012). Redox potential We measured redox potential of 20 plots within the experiment on 18 June, 2013 using a WTW Weilheim 330 handheld pH/mV meter (ORP METTLER TOLEDO). Conditions at the site were strongly anoxic at this point (18 days after the flooding began), and thus redox potential measurements were unreliable and impossible to obtain in many of the most severely flooded plots. We therefore do not include redox potential directly in any of our models, but report that conditions at the site were consistently anaerobic (ranging from −121 to 193 mV; ref. 28 ). Soil microbial biomass and soil nitrate concentrations Soil microbial biomass (μg Cmic per g dry soil) was measured in May 2010, April 2011, April 2012, May 2013, July 2013, and September 2013. Microbial biomass was measured by sampling five randomly located 2 × 5 cm (depth) soil cores in each plot. Soil was then pooled and sieved to remove visible roots and larger soil animals. Substrate–induced respiration was obtained using an O 2 –microcompensation apparatus [29] and used to calculate soil microbial biomass C. Soil nitrate concentration (μg NO 3 per g dry soil) was measured in September 2010, September 2011, September 2012, and October 2013. Soil nitrate was obtained by randomly sampling five soil cores per plot (2 × 15 cm depth), pooling samples, and conducting an extraction with 1 M KCl (5 g soil per 50 ml KCl). Nitrate concentrations were analyzed colorimetrically using a Continuous Flow Analyzer (AA3, SEAL, Norderstedt, Germany). Statistical model These models account for spatial autocorrelations associated with measurements taken within the same block of the field site (block i ) and temporal autocorrelation associated with taking multiple measurements on the same plots over time (plot ij ): y = μ + β 1 SpRich ij + β 2 FloodSeverity ij + β 3 Time ij + β 4 SpRich ij FloodSeverity ij + β 5 SpRich ij Time ij + β 6 FloodSeverity ij Time ij + β 7 SpRich ij FloodSeverity ij Time ij +Block i +Plot ij . How to cite this article: Wright, A. J. et al . Flooding disturbances increase resource availability and productivity, but reduce stability in diverse plant communities. Nat. Commun. 6:6092 doi: 10.1038/ncomms7092 (2015).